Ballistic-like supercurrent in suspended graphene Josephson weak links The interplay of the massless Dirac fermions in graphene and the Cooper pair states in a superconductor has the potential to give rise to exotic physical phenomena and useful device applications. But to date, the junctions formed between graphene and superconductors on conventional substrates have been highly disordered. Charge scattering and potential fluctuations caused by such disorder are believed to have prevented the emergence or observation of new physics. Here we propose to address this problem by forming suspended graphene–superconductor junctions. We demonstrate the fabrication of high-quality suspended monolayer graphene–NbN Josephson junctions with device mobility in excess of 150,000 cm 2 per Vs, minimum carrier density below 10 10 cm −2 , and the flow of a supercurrent at critical temperatures greater than 2 K. The characteristics of our Josephson junctions are consistent with ballistic transport, with a linear dependence on the Fermi energy that reflects of linear dispersion of massless Dirac fermions. Graphene is a promising material for building superconducting devices. In ambient environment, it is inert against surface oxidation which makes it relatively easy to fabricate transparent interface with the superconducting electrodes. The low-charge carrier density inside graphene is easily tunable using electric field effect, adding a useful knob for studying the density/energy dependence of the physical properties of the system. Moreover, the quasiparticles in graphene are Dirac fermions with linear energy dispersion and a vanishing density of state at the Dirac point where the conduction and valence bands touch. Such electronic structure offers intriguing new physics in superconducting proximity effect [1] , [2] , [3] , [4] , [5] . In particular, at close vicinity to the Dirac point, the specular Andreev reflection [1] and a supercurrent supported [2] by evanescence modes have been theoretically predicted. Away from the Dirac point, the intrinsic ballistic Josephson current depends linearly on the Fermi energy [2] . From the practical point of view, the high mobility of the charge carriers in graphene allows a decent magnitude of supercurrent in the superconducting weak links. The tunability of the supercurrent through electric field gating suggests the potential applications in the graphene–superconductor devices [6] , [7] , [8] , [9] . Graphene Josephson devices were first demonstrated in graphene–-Al junctions [3] , [4] that were characterized at millikelvin temperatures. More recently, graphene Josephson devices have been studied using superconducting contacts with higher transition temperatures, such as Pb [10] , Nb [11] , [12] and ReW [12] . Up to the present, the reported graphene–superconductor devices have been fabricated on SiO 2 . A serious limitation of the devices is that the substrates induce severe disorders from the roughness and charge traps. Such disorders limit the devices to be within the diffusive regime with a typical electron mean free path of a few tens of nanometres. Random doping from the substrate creates the electron-hole puddles [13] and limits the minimum carrier density to ~10 11 cm −2 , which corresponds to large potential fluctuations of >30 meV. This hinders the tuning of the Fermi energy of graphene to the close vicinity of the Dirac point. To date, there have been two major approaches for fabricating high-mobility graphene devices: by suspending graphene [14] , [15] and by placing graphene on a h-BN substrate [16] . Compared with the reported graphene-hBN devices, suspended graphene devices are restricted in the channel size and device geometry, and yet they give the highest device mobility with the lowest potential fluctuations (minimum residue carrier density). The maximum mobility achieved in the suspended graphene junctions is much higher than 200,000 cm 2 per Vs for a minimum carrier density achievable at ~10 9 cm −2 . For the Josephson junction devices, only simple two-terminal geometry with short channel length is necessary. Therefore, suspended graphene technique is in principle suitable. Here we demonstrate the fabrication and characterization of the high-quality suspended monolayer graphene–NbN Josephson junctions that have device mobility greater than 150,000 cm 2 per Vs, with minimum carrier density below 10 10 cm −2 and a formation of supercurrent at temperature above 2 K. The devices have exhibit ballistic-like Josephson currents that depend linearly on the Fermi energy of graphene, which is consistent with the theoretical prediction based on the linear energy dispersion of the Dirac electrons. Device fabrication Fabrication of the suspended graphene–superconductor junction has two main challenges: The first is to make the suspended structure without wet chemical etching (typically requires hydrofluoric acid or buffered oxide etchant [14] , [15] , which attacks most superconductors), and the second is to produce highly transparent graphene–superconductor contacts. We have developed a single-lithography fabrication technique in which graphene is mechanically exfoliated on top of a polymethyl methacrylate (PMMA) resist spacer on a SiO 2 substrate. A methyl methacrylate (MMA) resist layer is then spin-coated for contact definition. By the electron beam dose control, we expose and develop the 3-dimensional surface profile that forms the suspended graphene structure after the metallization and lift-off in solvents (see Supplementary Note 1 ). To fabricate the transparent graphene–superconductor contacts, NbN is reactively sputtered using Nb target in Ar/N 2 plasma. Careful adjustments of the N 2 and Ar gas partial pressure, the DC sputtering power and the sample-target distance are conducted to minimize the stress, as well as optimizing the transition temperature of the thin film (see Supplementary Note 2 ). Before the sputtering of NbN we e-beam evaporate Ti/Pd bilayer on graphene to create high transparency and to reduce the damage from energetic ions. The Ti layer serves the purpose of enhancing the adhesion of NbN film, and Pd is used to prevent the reaction of the Ti with the N 2 plasma. In the reactive sputtering, ~70 nm-thick NbN is coated to form the contacts. This simple technique allows the fabrication of the suspended graphene junctions, with arbitrary metal contacts and on arbitrary substrates. Comparing with similar Au/Ti-contact devices fabricated by wet etching methods [14] , [15] our method yields high-quality suspended graphene Au/Ti junctions with a maximum mobility >200,000 cm 2 per Vs at a minimum carrier density of ~3 × 10 9 cm −2 . Well-defined integer quantum Hall plateaus of ν =2, 6, 10, 14 can readily be observed in a low magnetic field of 0.5 T at 4.2 K ( Supplementary Fig. S2 ). Device characterization Combining the wet-etching-free suspending techniques and the NbN deposition, we fabricated the monolayer graphene–NbN weak link ( Fig. 1e ) with a width of 1.8 μm and a length of 0.5 μm. The device was cooled in a cryostat for electrical characterizations. The as-fabricated suspended graphene device typically does not show good quality before the current annealing treatment ( Fig. 2a Inset). A large current (~0.3–0.4 mA μm −1 ) annealing was conducted to clean the graphene channel in situ. The NbN leads became superconducting below the transition temperature of T c ~12 K (see Supplementary Fig. S3 ), and we observed a decreasing weak-link resistance with decreasing temperature. To monitor the effect of large current annealing on the graphene–NbN interface, we measure the Andreev reflection features after each high-current annealing ramp. Figure 2b shows the typical differential resistance (d V /d I ) versus bias voltage, measured at 4.2 K. The features of the multiple Andreev reflections are clearly observable for the as-fabricated device. 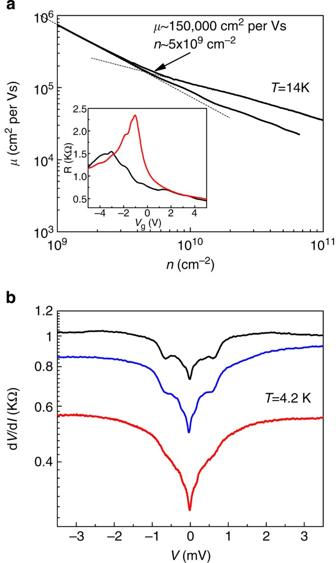Figure 2: Effect of current annealing. (a) Carrier density dependence of mobility after current annealing. The low carrier density regime whereμ~1/n(hence, σ=nμe~const) is within the electron-hole ‘puddles’. Above a minimum carrier density of 5 × 109cm−2, where the mobility switches to, the carrier density can be considered uniform. The two curves correspond to the electron branch (higher mobility) and the hole branch (lower mobility). (a) Maximum mobility of ~150,000 cm2per Vs was measured on this device just outside the electron-hole puddles. Inset: Comparison of resistance versusVgbefore (black) and after (red) current annealing, measured atT>Tc. (b) Evolution of the Multiple Andreev reflection characteristics before, during and after current annealing. We notice that the superconducting gap (2 Δ ~1 meV) appears to be rather strongly suppressed compared with the estimation from the transition temperature ( Δ (0)=1.764 k B , T c ~1.8 meV). The gap reduction had been previously observed in Josephson weak links, including graphene-based Josephson weak links [17] . Pd appears to have significant effect in reducing the gap size [18] . Qualitatively the gap reduction can be understood as due to the decreasing of the order parameter across the Ti/Pd buffer layers. At near-zero bias a sharp dip can be seen corresponding to the development of the supercurrent. Although current annealing, the device is Joule-heated under the increasingly higher current. The mobility of the device increases, while the ratio of the zero-bias resistance to the normal state resistance decreases, indicating the high transparency of the graphene–NbN interface. The d V/ d I versus V b curve develops into a ‘V’ shape after the annealing, and the oscillatory multiple Andreev reflection feature before current annealing becomes less pronounced. The observed changes in the bias voltage dependence of the sub-gap differential resistance from current annealing are qualitatively consistent with the reduction of scattering centres inside the graphene weak link and possibly at the interface. It has been shown theoretically [19] that, for a single quantum channel, the oscillatory features associated with the multiple Andreev reflections are absent unless when enhanced by a finite reflection probability. For graphene with two dimensional modes, due to the finite reflection probability properties resulting from the mismatch between the band structures of graphene the contacts, one expects oscillatory multiple Andreev reflection behaviour. 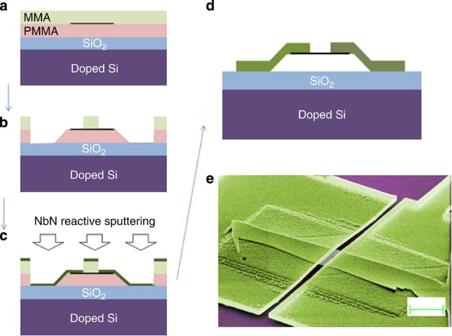Nevertheless, as the modes transmit current independently [20] in the multi-mode junctions, one can expect that the oscillatory amplitude from the multiple Andreev reflections reduces for near ballistic junctions, with the reduction of scattering and hence the enhancement of transmission probability. Figure 1: Fabrication of suspended graphene–NbN Josephson junction. (a) Graphene is mechanically exfoliated on top of PMMA resist and then spin-coated with MMA resist. (b) E-beam lithography on the resists opens windows on the contact areas. (c) NbN is deposited through reactive DC sputtering of Nb in Ar and N2plasma. (d) Lift-off in solvents reveals the suspended graphene–NbN structure. (e) False-color scanning electron microscope (SEM) image of a graphene–NbN Josephson junction. Here the junction width isW=1.8 μm, and length isL=0.5 μm. Scale bar, 2 μm. Figure 1: Fabrication of suspended graphene–NbN Josephson junction. ( a ) Graphene is mechanically exfoliated on top of PMMA resist and then spin-coated with MMA resist. ( b ) E-beam lithography on the resists opens windows on the contact areas. ( c ) NbN is deposited through reactive DC sputtering of Nb in Ar and N 2 plasma. ( d ) Lift-off in solvents reveals the suspended graphene–NbN structure. ( e ) False-color scanning electron microscope (SEM) image of a graphene–NbN Josephson junction. Here the junction width is W =1.8 μm, and length is L =0.5 μm. Scale bar, 2 μm. Full size image Figure 2: Effect of current annealing. ( a ) Carrier density dependence of mobility after current annealing. The low carrier density regime where μ ~1/ n (hence, σ= nμe ~const) is within the electron-hole ‘puddles’. Above a minimum carrier density of 5 × 10 9 cm −2 , where the mobility switches to , the carrier density can be considered uniform. The two curves correspond to the electron branch (higher mobility) and the hole branch (lower mobility). ( a ) Maximum mobility of ~150,000 cm 2 per Vs was measured on this device just outside the electron-hole puddles. Inset: Comparison of resistance versus V g before (black) and after (red) current annealing, measured at T > T c . ( b ) Evolution of the Multiple Andreev reflection characteristics before, during and after current annealing. Full size image After the current annealing, the maximum mobility of the device shown here reaches for the electron branch, with a minimum carrier density of ~5 × 10 9 cm −2 ( Fig. 2a ) and a Dirac point gate voltage of V D =−1.03 V. In calculating the carrier density ( C/A being gate capacitance per area), we consider the vertical geometry of the suspended structure on top of SiO 2 . As a result, the gate capacitance per area is , where and . Here ε SiO2 =4 is the dielectric constant of SiO 2 , d SiO 2 =285 nm is the thickness of SiO 2 , ε vacuum =1 is the dielectric constant of vacuum, and d vacuum =250 nm is the height with which graphene is suspended over SiO 2 (estimated from the thickness of the PMMA spacer). Between the electron and the hole branches, we observed an asymmetry with the hole branch showing higher resistance and weak oscillatory (Fabry–Pérot) gate voltage dependence. Such asymmetry behaviour is commonly observed in clean short-channel graphene devices [15] , [21] . Its presence has been studied theoretically to be due to the charge-transfer at the metal-graphene interface, which induces asymmetric potential profiles near the contacts for electron and hole doping. Here we focus our discussion on the electron branch which has shown higher mobility. The carrier mobility in this electron branch follows μ ~ n −1/2 ~1/ E F (that is, conductivity σ ~ n 1/2 ~ E F ), which is consistent with ballistic transport in a two-terminal device [22] , [23] . The mean free path for electron branch is estimated to be and is found to be roughly V g -independent throughout the range of the gate voltage applied, consistent with two-terminal ballistic transport in graphene. Josephson current A clear evidence of the Josephson current is observed in the sample cooled to below 3 K. The IV characteristics of the junction measured at T =2.2 K is shown in Fig. 3b . By changing the gate voltage we can tune the magnitude of the supercurrent. Fig. 3b shows the temperature dependence of the Josephson current measured at V g =5 V. With increasing temperature the supercurrent decreases and a zero-bias resistance becomes evident at T ~3 K. Based on the junction parameters, we estimate (for V g =5 V, R N =500 Ω, I c ~100 nΑ, C ~10 −12 F) the Stewart–McCumber parameter to be . (Here the value of C is estimated from the capacitance between the source and drain pads coupled from the conducting back gate [3] ). This indicates the device to be underdamped based on the resistively and capacitively shunted junction (RCSJ) model [24] , in which the Josephson weak link is described by a simple circuit consisting of a ‘intrinsic’ Josephson junction, a capacitor, and a resistor in parallel. In a current driven Josephson weak link, the RCSJ can be described by equation: , where I is the driving current, φ the phase difference between the two superconducting contacts, R the normal state resistance, C the junction capacitance and I c the intrinsic Josephson current. Here we used the approximation that the current–phase relation is sinusoidal, while in the actual devices the current–phase relation is skewed [9] , [25] , [26] . Such sinusoidal approximation is justified since the error is smaller than ~5% (see Supplementary Note 3 ). For an underdamped Josephson weak link, the RCSJ model yields IV characteristics which are highly hysteretic. On the other hand, the IV curves at the temperatures and gate voltages studied here are non-hysteretic and the transitions from Josephson current to the normal state are gradual. The observed smoothened IV curves can be understood by considering the noise parameter that describes the ratio of the thermal energy to the Josephson coupling energy: . For a critical current of ~100 nA, this gives Γ ~1. It has been demonstrated in diffusive graphene Josephson weak links at millikelvin temperatures (when Γ <<1) that the supercurrent is reduced through a premature switching process [3] , [17] , [27] . For stronger thermal fluctuation, however, phase diffusion dominates and causes a finite voltage in the supercurrent regime as well as gradual switching [28] , [29] . 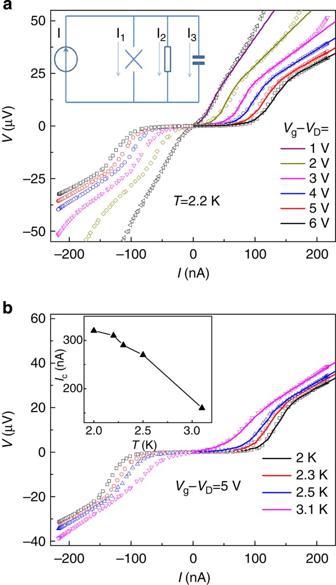Figure 3: Supercurrent in suspended graphene–NbN Josephson junction. (a) Current-voltage characteristics at various gate voltages measured atT=2.2 K. Symbols are experimental data and solid lines are corresponding fittings from numerical simulations. Inset: the RCSJ model. (b) Temperature dependence of the supercurrent, measured at a gate voltage ofVg=5 V. Symbols are experimental data and solid lines are corresponding fittings from numerical simulations. Figure 3: Supercurrent in suspended graphene–NbN Josephson junction. ( a ) Current-voltage characteristics at various gate voltages measured at T =2.2 K. Symbols are experimental data and solid lines are corresponding fittings from numerical simulations. Inset: the RCSJ model. ( b ) Temperature dependence of the supercurrent, measured at a gate voltage of V g =5 V. Symbols are experimental data and solid lines are corresponding fittings from numerical simulations. Full size image To our knowledge, there is no analytical solution to the IV characteristics of a Josephson weak link under the strong thermal fluctuation with arbitrary β c . To fit the IV curves and obtain the value of the intrinsic Josephson current I c , we carry out a numerical simulation that solves the RCSJ model under a DC driving current in parallel with a Johnson–Nyquist noise current. To ensure the accuracy of our simulation, we compute the temperature dependence of the IV curves for the extreme case of a strongly overdamped junction where analytical solution was obtained using the Ambegaokar–Halperin model [29] (see Methods). There our calculation precisely overlaps with the analytical solution. We also compared our calculations with the previous numerical study of the RCSJ model with noise in both overdamped and underdamped regimes, and obtained precise quantitative agreement (see Method and Supplementary Note 3 ). We then apply the calculation to our data. In Fig. 3 , the simulated IV curves are compared with the experimental data and quantitative agreements have been reached. In the fittings, the normal resistance outside the supercurrent regime is directly taken from the slope of the IV curves, which has temperature-dependent values that are smaller than the R N values measured just above T c . We use the effective resistance above the switching (instead of R N ), because, as a circuit model, the RCSJ model by itself does not contain the physics of the superconducting proximity effect and the value of R in the model simply corresponds to the DC resistance of the junction in absence of a supercurrent. Due to the Andreev reflection enhancement of conductance, the value of R is smaller than that of R N measured at above T c (or outside the superconducting gap), and is temperature dependent. Although exactly what resistance should be used for calculating the Josephson dynamics is not settled by a rigorous quantitative theory, qualitatively it is reasonable to use the effective resistance above the switching current, because the phase is a macroscopic variable, and its dynamics is affected by the total junction response in which one cannot separate the quasiparticle current from Andreev current. The capacitance used in our calculations is fixed to 1.4 pF. For noise calculations, we used the temperature T = T EM + T b , where T b is the actual bath temperature and T EM ~0.4 K is an estimated equivalent noise temperature of the electro-magnetic environment. The only free parameter used in the fittings is the Josephson current. From this we obtain the temperature and the gate-voltage dependence of the Josephson current I c , shown in Figs 3 and 4 . The Josephson current decreases with increasing temperature and with increasing normal resistance tuned by the gate voltage. 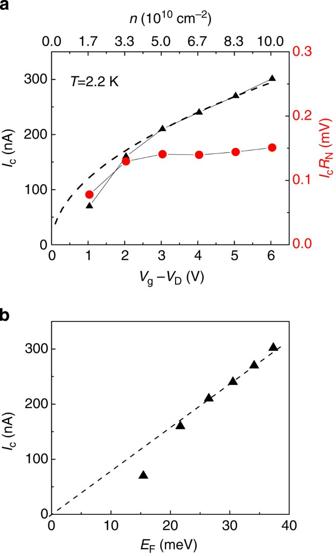Figure 4: Tuning of the intrinsic Josephson current. (a) Dependence of Josephson current (left axis) andIcRNproduct (right axis) on gate voltageVg−VD(VDbeing the gate voltage at the Dirac point) and carrier density. The dotted line is a guide to the eyes, which shows a square-root carrier density dependence. (b) Dependence of Josephson current on Fermi energy. At large Fermi energies, the dependence is linear. Dotted line is given as a guide to the eyes for the linear dependence. Figure 4: Tuning of the intrinsic Josephson current. ( a ) Dependence of Josephson current (left axis) and I c R N product (right axis) on gate voltage V g − V D ( V D being the gate voltage at the Dirac point) and carrier density. The dotted line is a guide to the eyes, which shows a square-root carrier density dependence. ( b ) Dependence of Josephson current on Fermi energy. At large Fermi energies, the dependence is linear. Dotted line is given as a guide to the eyes for the linear dependence. Full size image An interesting feature of the intrinsic Josephson current is that, except for near the Dirac point, the Josephson current shows a linear dependence on the Fermi energy, as shown in Fig. 4b . This is in qualitative agreement with the theoretical prediction for a ballistic graphene Josephson weak link [2] . At large Fermi energies, such linear dependence can be related to the combination of a constant I c R N product and a linear Fermi energy dependence of the normal conductance, which is a signature of the ballistic transport. The observed I c R N product is roughly independent of the gate voltage except near the Dirac point. This is significantly different from what one would expect in a diffusive SNS long junction, where the I c R N depends on the mean free path [30] that is normally V g -dependent [31] , [32] . Although for a highly disordered short junction, the I c R N product is also expected to be mean free path-independent [30] , such devices should have a mean free path which is much smaller than the effective junction length, which is not the case observed here. In Fig. 4a , significant decrease in the I c R N product is evident for V g − V D ≤2 V corresponding to low carrier density n ≤3 × 10 10 cm −2 , well beyond the low-density limit for any on-substrate devices as a result of strong potential fluctuations. The observed decrease in the I c R N product qualitatively agrees with the expectation of the quasi-diffusive transport of the evanescence modes near the Dirac point, predicted by the theory of the Josephson effect in ballistic graphene junctions [2] . On the other hand, at our base temperature of 2 K, the IV curves exhibit an Ohmic behaviour for low carrier density n <10 10 cm −2 as the Josephson energy decreases and the noise parameter becomes Γ ~1. In this low-density regime at the close vicinity of the Dirac point, lower temperatures is required to accurately measured supercurrent. Compared with the theoretical predictions on ideal-wide ballistic Josephson weak links [2] , [9] , where , the value of the I c R N product obtained from our measurements, , is much smaller. Such discrepancy may be attributed to the imperfect graphene–superconductor interface, and the relatively high-measurement temperature. Finally, to study the stability of the suspended graphene–NbN devices, we thermal cycle our samples by warming it to the room temperature and re-cooling it to repeat the measurements. The devices showed an excellent thermal stability and the quality was unaffected by the thermal cycling. The devices were examined after being kept in raw vacuum (~100 mTorr) for ~ 1 month and no sign of obvious aging was observed after the idling time. The excellent characteristics of the suspended graphene Josephson junction, including ultrahigh mobility, low potential fluctuations, transparent interface and stability, open the door to a wide range of research opportunities allowing one to study the interplay between magnetotransport, superconducting proximity effect and nanoelectromechanical properties in graphene. Potentially these may lead to better understanding the fundamental physics of the 2D Dirac fermion system as well as developing of novel device concepts. Device fabrication To fabricate the suspended graphene devices, we follow the procedure illustrated in Fig. 1 . First, we coat a Si/SiO 2 substrate with a PMMA 950 K A4 resist spun at 3,000 r.p.m. The thickness of the resist spacer (~250 nm) determines the distance between the suspended graphene channel and the surface of SiO 2 (see Supplementary Note 1 ). Graphene is then mechanically exfoliated on the PMMA film, followed by spin coating of a MMA EL8.5 copolymer resist for the contact definition ( Fig. 1a ). By the electron beam dose control, we expose and develop the three-dimensional surface profile that forms a suspended structure after the metallization and lift-off. A low E-beam dose is used for the exposure of the contact area on top of graphene, and a high dose is used for the surrounding areas of the contacts. Consequently, after developing process, both of the exposed MMA/PMMA layers are removed from the substrate, while only the MMA will be removed from the graphene contact area ( Fig. 1b ). It should be noted that for the E-beam exposure an accurate dose control is not necessary; because as long as the dose is sufficiently high to expose through the MMA layer, the graphene flake itself will block the developer, preventing the overdeveloping of the PMMA underneath. This gives a high fabrication yield at relatively mild demands on the exposure parameters. As the graphene-covered plateau is high above the substrate surface, in order to ensure the continuity of the metallic contacts we apply a gradual exposure dose change between the high-dose and low-dose regions. Following the E-beam lithography process, the sample is metalized in a high-vacuum chamber with a base pressure <2 × 10 −8 Torr, equipped with a four-pocket e-beam evaporator and a DC magnetron sputtering source. We reactively sputter a superconducting NbN film using Nb target in Ar/N 2 plasma. Careful adjustments of the N 2 and Ar gas partial pressure, the DC sputtering power and the sample-target distance are carried out to minimize the stress, as well as optimizing the transition temperature of the thin film. In addition, before the sputtering of NbN, we e-beam pre-evaporate a buffer layer of Ti (~2 nm)/Pd (~1.5 nm) to create a highly transparent interface between graphene and the NbN contacts and to reduce damage from energetic ions. The Ti layer serves the purpose of improving the adhesion of the contact material with graphene and the Pd layer prevents undesirable reaction of the Ti with the N 2 plasma. Immediately after E-beam evaporation of the Ti/Pd bilayer, we sputter NbN without breaking the vacuum ( Fig. 1c ). To start the reaction, the pressures of Ar (6.7 mTorr) and N 2 (0.9 mTorr) are independently controlled by adjusting their corresponding flows. The sample is located 10 cm away from a 3′′ Nb target. A constant power of 470 W is maintained during the sputtering. After the plasma is started, we carried out 80 s pre-sputtering, followed by sputtering of 70 nm-thick NbN onto the sample at the deposition rate of ~1 nm s −1 . The lift-off is performed in acetone after the metallization. The sample is immersed in two successive acetone baths at 80 °C. Then, although the sample is kept wet, it is transferred and rinsed in a room temperature IPA Bath. Finally, the sample is quickly moved into a hot IPA bath, which is slightly below the boiling point, and then directly taken out to be dried in air ( Fig. 1d ). Numerical calculation of the RCSJ model We assume that our devices can be described by the resistively and capacitively shunted Josephson junction (RCSJ) model (see inset of Fig. 3a ). The driving current (given) split into three flowing through the ‘pure’ Josephson junction, the resistor and the capacitor. Hence; Here, i = I / I c =( I app + I noise )/ I c consists of an applied current and a noise current. To solve the equation numerically, we change the differential equation to difference equation: d t →Δ t dt and equation (1) changes to: here A =ħ/ 2eRI c , B =ħC/ 2eI c , and Δ t is chosen to be much (~1,000 times) smaller than the period of the Josephson oscillations. Given a initial condition of φ 1 , φ 2 and the normalized current, i ( t ), we can solve for φ ( t ). Then, from φ ( t )we can calculate the averaged DC voltage: For I noise we used the Johnson noise current generated as a Gaussian white noise and related to the temperature by , where f is the bandwidth used in our simulation. For each generated Johnson noise, we calculate an IV curve based on the above method. The IV curves are averaged 100 times over randomized Johnson noise currents. The final results are compared with the experimental data. To ensure the reliability of the simulations, we compare our simulation results for the case of strongly underdamped junctions with the Ambegaokar–Halperin model [27] , [29] , as shown in Supplementary Fig. S4 . The simulation results quantitatively agree with the model. We also compared our simulation with the previous study in the underdamped regime. Supplementary Fig. S4 shows the quantitative agreement between the results obtained by R.F. Voss [33] and that from our calculations. How to cite this article: Mizuno, N. et al. Ballistic-like supercurrent in suspended graphene Josephson weak links. Nat. Commun. 4:2716 doi: 10.1038/ncomms3716 (2013).